An integrated approach to realizing high-performance liquid-junction quantum dot sensitized solar cells Solution-processed semiconductor quantum dot solar cells offer a path towards both reduced fabrication cost and higher efficiency enabled by novel processes such as hot-electron extraction and carrier multiplication. Here we use a new class of low-cost, low-toxicity CuInSe x S 2− x quantum dots to demonstrate sensitized solar cells with certified efficiencies exceeding 5%. Among other material and device design improvements studied, use of a methanol-based polysulfide electrolyte results in a particularly dramatic enhancement in photocurrent and reduced series resistance. Despite the high vapour pressure of methanol, the solar cells are stable for months under ambient conditions, which is much longer than any previously reported quantum dot sensitized solar cell. This study demonstrates the large potential of CuInSe x S 2− x quantum dots as active materials for the realization of low-cost, robust and efficient photovoltaics as well as a platform for investigating various advanced concepts derived from the unique physics of the nanoscale size regime. Solar cells utilizing colloidal quantum dots (QDs) as the light-absorbing material have seen rapid advances in recent years [1] from the first certified power conversion efficiency (PCE) of 3% reported in 2010 (ref. 2 ) to >7% last year [3] . These high-performance certified devices have used PbS QDs, and are notable for their low cost of fabrication and ability to efficiently harvest the near-infrared portion of the solar spectrum. Furthermore, the measurement of external quantum efficiencies (EQEs) above 100% using PbSe QDs [4] demonstrates the potential of these devices for surpassing the Shockley–Queisser limit [5] by employing carrier multiplication. Although recent progress in QD photovoltaics (PVs) based on Pb X ( X =S, Se) QDs is promising, major challenges to reaching commercializable efficiencies remain. The primary factor limiting performance of these devices is high recombination losses in the active layer due to presence of charge traps that originate from surface states. This results in short diffusion lengths for minority carriers [6] in QD solids and ultimately limits the thickness of the active layer to <500 nm ( Fig. 1a ), which is insufficient for complete absorption of incident photons. Furthermore, the p–n heterojunction architecture requires fine control over carrier doping in order to tune the depletion width, which is another outstanding challenge [7] , [8] , [9] . The high atomic fraction of toxic lead atoms and the generally poor stability of Pb X QDs under ambient conditions further complicate commercialization of this emerging technology, although PbS QD solar cells have been demonstrated with 1,000 h stability under continuous illumination in air [2] . 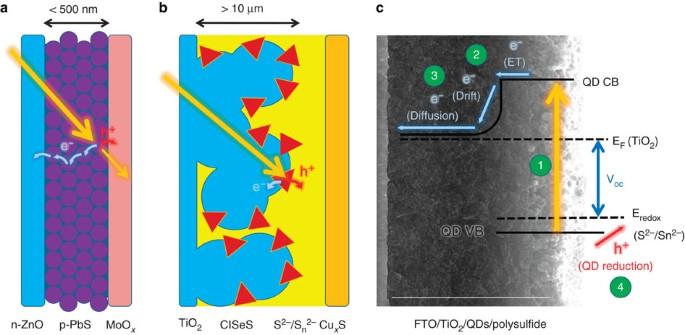Figure 1: Working principles of colloidal QD solar cells. (a) Schematic of a typical thin-filmp–njunction QD PV (PbS QDs are purple circles, the contacts are omitted); high recombination losses due to the long paths for minority carriers to reach the electrode ultimately limit the thickness of the QD layer. (b) Schematic of the QDSSC architecture (CISeS QDs are red triangles, the contacts are omitted) that avoids QD-to-QD carrier transport completely, and benefits from more complete light absorption and a modular design. See Methods andSupplementary Informationfor the details of device design and fabrication. (c) QDSSC photoanode (SEM (scanning electron microscope) cross-sectional image) along with a schematic band structure (VB and CB are valence and conduction bands, respectively) and the depiction of various steps of the light conversion process: (1) generation of an excited electron (e−)—hole (h+) pair by an absorbed solar photon, (2) electron transfer (ET) to TiO2, (3) electron drift followed by diffusion within the TiO2anode, (4) hole transfer to (QD reduction by) polysulfides in the electrolyte (not necessarily after steps 2 or 3) and (5) hole collection by (oxidation of) the CuxS electrode (not shown);EFis the Fermi level of the TiO2anode andEredoxis the electrolyte redox potential. Scale bar, 10 μm. Figure 1: Working principles of colloidal QD solar cells. ( a ) Schematic of a typical thin-film p–n junction QD PV (PbS QDs are purple circles, the contacts are omitted); high recombination losses due to the long paths for minority carriers to reach the electrode ultimately limit the thickness of the QD layer. ( b ) Schematic of the QDSSC architecture (CISeS QDs are red triangles, the contacts are omitted) that avoids QD-to-QD carrier transport completely, and benefits from more complete light absorption and a modular design. See Methods and Supplementary Information for the details of device design and fabrication. ( c ) QDSSC photoanode (SEM (scanning electron microscope) cross-sectional image) along with a schematic band structure (VB and CB are valence and conduction bands, respectively) and the depiction of various steps of the light conversion process: (1) generation of an excited electron (e − )—hole (h + ) pair by an absorbed solar photon, (2) electron transfer (ET) to TiO 2 , (3) electron drift followed by diffusion within the TiO 2 anode, (4) hole transfer to (QD reduction by) polysulfides in the electrolyte (not necessarily after steps 2 or 3) and (5) hole collection by (oxidation of) the Cu x S electrode (not shown); E F is the Fermi level of the TiO 2 anode and E redox is the electrolyte redox potential. Scale bar, 10 μm. Full size image An alternative device architecture for utilizing QD absorbers is the liquid-junction-sensitized solar cell pioneered by O’Regan and Grätzel [10] , [11] . In sensitized PVs, a meso-porous (mp) TiO 2 anode decorated with a narrow-gap absorber is contacted by an electrolyte solution that provides a conductive pathway to a metal or semiconductor cathode ( Fig. 1b ). This architecture avoids inefficient QD-to-QD carrier transport by employing discrete interfacial charge-transfer steps in which a photo-excited electron transfers from the QD to TiO 2 , while the remaining hole is reduced by the electrolyte ( Fig. 1c ). Traditionally this device architecture has utilized dye molecules as light absorbers/sensitizers [10] . The best dye-sensitized solar cells (DSSCs) reach efficiencies in excess of 10%, with a current record of 12.3% [12] . However, despite the large promise, widespread application of DSSCs is complicated by inherent limitations of the dyes themselves, which usually contain low-abundance elements such as ruthenium, have limited absorption bandwidth and suffer from photo-bleaching and poor long-term chemical stability, particularly under strong illumination [13] . To circumvent the drawbacks of dyes, several groups have explored replacing them with QDs [14] , [15] , [16] , [17] , [18] . The investigated approaches include infusion of pre-synthesized colloidal QDs into the mp-TiO 2 (refs 17 , 19 , 20 , 21 ) and direct growth of semiconductor clusters within the matrix [14] , [15] , [16] , [22] . This latter method was used to achieve the highest reported (yet uncertified) efficiency of 5.6% in structures comprising PbS:Hg QDs deposited with a successive ionic layer adsorption reaction (SILAR) [23] . These devices however were highly unstable and degraded over a period of minutes, meaning that accurate characterization of their performance was extremely difficult due to transient changes in device characteristics. In principle, colloidal QD sensitizers can have several advantages over SILAR-deposited QDs that arise from the ability to synthesize them under optimal conditions. This allows for much better control over size, composition [20] , shape and heterostructuring, and generally results in QDs with improved crystallinity and stability. Indeed, we recently reported proof-of-principle sensitized solar cells utilizing colloidally synthesized CuInSe x S 2− x (CISeS) QDs [24] . This previous work was a synthesis-focused effort on optimizing QD structural parameters for achieving more complete coverage of the solar spectrum, enhancing QD surface chemistry for multi-day stability and maximizing the loading of QDs into the pores of the TiO 2 matrix. In the course of this study, we determined that the optimal QD parameters corresponded to the CuInSe x S 2− x alloy with x =1.4 and an averaged QD size of ~4.5 nm (in these pyramidal QDs, size is the measured length from an apex to the midpoint of the opposing edge of the triangular projections observed in TEM images). Without exploring the parameter space extensively, we also noted that exposing the QDs to Cd-oleate could be beneficial to QD-sensitized solar cell (QDSSC) performance. With an energy gap ( E g ) of ~1.3 eV, the optimized CISeS QDs allowed for ~100% absorption and a maximum external quantum efficiency (EQE) of ~45% (at 3 eV) and an overall uncertified PCE of 3.5% in the best devices. [24] QDSSCs based on CuInS 2 QDs (without Se) have also been reported in recent years with uncertified efficiencies as high as 4.7% [25] , [26] , [27] ; however, the maximum photocurrent achievable for this material is roughly the same as for CdSe QDs due to the relatively large bulk band-gap. In the present report we reveal a crucial effect of CISeS QD surface properties on device performance. Specifically, by utilizing inorganic passivation of the QDs with partial cation exchange using Zn 2+ or Cd 2+ ions prior to sensitization, we suppress non-radiative recombination, which otherwise can outcompete fairly slow (>5 ns) electron transfer into the mp-TiO 2 photoanode. Further, we demonstrate the importance of recapping with short ligands in order to achieve efficient sensitization via direct attachment [28] . In addition, we optimize the electrolyte composition and reveal the critical importance of improved wetting through methanol addition for achieving high performance in these liquid-junction solar cells. We find that in addition to improving short-circuit current, tuning electrolyte composition allows us to reduce series resistance of the devices and thus increase the fill factor (FF). A further improvement in FF is obtained via the utilization of a meso-textured, high-surface-area Cu x S cathode. These coordinated efforts to understand and optimize the various stages of the photoconversion process have allowed us to achieve a record-long stability of several months under ambient conditions, the first-ever certified efficiency of 5.1% and a champion efficiency of 5.5%, which are record values for this emerging class of PV devices and among the highest reported for QD PVs [29] . Synthesis and surface modification of CISeS QDs The synthesis of colloidal CISeS QDs uses 1-dodecanethiol (DDT) as an effective yet low-cost solvent, ligand and sulphur precursor; controlled amounts of trioctylphosphine selenide (TOP-Se) are added to produce an alloy of reduced band-gap [24] , [30] . This synthetic approach results in pyramidally shaped CuInSe x S 2− x QDs (inset in Fig. 2a ) with x as high as ~1.6 (that is 80% Se anions, as measured by inductively coupled plasma optical emission spectroscopy (ICP-OES)). Utilizing as-synthesized CISeS QDs results in relatively poor PV performance [24] , which is primarily due to significant non-radiative losses associated with surface traps [30] . To address this issue, following the synthesis of the QDs, we treat them with a zinc oleate (Zn-oleate) solution, which results in temperature-controllable Zn 2+ exchange with surface Cu 1+ and In 3+ , cations ( Supplementary Fig. S3 ). This procedure leads to a strong reduction in surface-related trap states as evidenced by an increase in the PL intensity ( Fig. 2a ) and a lengthening of the PL lifetime [31] , [32] . The suppression of non-radiative recombination also manifests as increased open-circuit voltage ( V oc , from 0.33 V for untreated QDs to as high as 0.54 V in the case of the optimal treatment with Zn 2+ at 100 °C) and short-circuit current ( J sc , from 2.7–6.0 mA cm −2 ) in devices ( Fig. 2b ; details can be found in Supplementary Table S2 ). However, as the degree of cation exchange increases, a maximum in device performance is quickly reached, and J sc then decreases even as the PL efficiency of QDs in solution increases ( Fig. 2a ). We attribute this phenomenon to partial suppression of electron transfer to TiO 2 by the increasingly thick Zn-rich surface layer, which serves as a barrier due to its significantly higher-lying conduction band [32] . This observation suggests that electron transfer to TiO 2 is fairly slow, especially after cation exchange with Zn 2+ , and is likely characterized by timescales comparable to those of exciton recombination in the QDs (tens of nanoseconds) [32] . 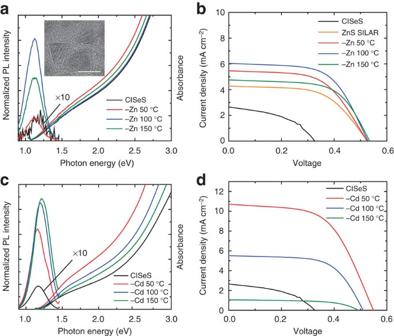Figure 2: Passivation of QD surfaces via cation exchange. (a) Absorption and photoluminescence (PL) spectra of the QDs before and after exposure to Zn-oleate at various temperatures after recapping with tert-butylamine (tBA). Inset: TEM image of 4.5 nm CuInSe1.4S0.6QDs. Scale bar, 5 nm. (b) Current density versus voltage characteristics for QDs with varying degrees of Zn-cation exchange, or with ZnS SILAR post-treatment of the QD-infused anode (orange line). (c) Absorption and PL spectra of the QDs before and after exposure to Cd-oleate and recapping with tBA. (d) Current density versus voltage characteristics for QDs with varying degrees of Cd-cation exchange controlled by reaction temperature. The photovoltaic performance properties related tobanddcan be found inSupplementary Tables S2 and S3. Figure 2: Passivation of QD surfaces via cation exchange. ( a ) Absorption and photoluminescence (PL) spectra of the QDs before and after exposure to Zn-oleate at various temperatures after recapping with tert-butylamine (tBA). Inset: TEM image of 4.5 nm CuInSe 1.4 S 0.6 QDs. Scale bar, 5 nm. ( b ) Current density versus voltage characteristics for QDs with varying degrees of Zn-cation exchange, or with ZnS SILAR post-treatment of the QD-infused anode (orange line). ( c ) Absorption and PL spectra of the QDs before and after exposure to Cd-oleate and recapping with tBA. ( d ) Current density versus voltage characteristics for QDs with varying degrees of Cd-cation exchange controlled by reaction temperature. The photovoltaic performance properties related to b and d can be found in Supplementary Tables S2 and S3 . Full size image In principle, treating the QDs in a colloidal suspension by cation exchange should be preferable to the commonly applied approach of depositing a thin layer of ZnS over the entire sensitized electrode by SILAR, since it enables greater flexibility in fabrication and characterization. On the other hand, ZnS deposited by SILAR may provide the benefits of inorganic passivation but without creating a barrier at the QD/TiO 2 interface [33] . In a comparison study, when a ZnS SILAR post-treatment (two monolayers) is applied to non-cation-exchanged CISeS QD-sensitized TiO 2 ( Fig. 2b , orange curve), the enhancement is similar yet slightly less pronounced than the colloidal/cation-exchange method. While we have observed real performance enhancement using cation exchange with Zn 2+ , the tendency of thicker Zn-rich surface layers to act as barriers to charge extraction is ultimately limiting. An isovalent alternative to Zn 2+ is Cd 2+ ; importantly, Cd(Se, S) has a lower-lying conduction band than Zn(Se, S) and therefore it might present a smaller (if any) barrier to electron transfer. We observe that the effect of cadmium oleate (Cd-oleate) exposure on CISeS QDs’ optical properties is approximately the same as with Zn-oleate ( Fig. 2a ) [24] : absorption remains essentially unchanged, while the PL intensities ( Fig. 2c ) and lifetimes dramatically increase. However, analysis of the composition with ICP-OES ( Supplementary Fig. S3 ) indicates that Cd-oleate is more reactive towards CISeS QDs at low temperature and results in a more aggressive exchange of cations. Comparing the performance of QDSSCs made from QDs treated with Zn-oleate ( Fig. 2b ) and Cd-oleate ( Fig. 2d ) at various temperatures, we find that while Zn-treated QDs (PCE of 1.91%) show a significant improvement over untreated QDs (0.38%), Cd treatment produces even a greater enhancement in the PV performance (3.34%). The best devices incorporated CISeS QDs treated at 50 °C, which corresponded to the mildest exposure to Cd 2+ ions with a resulting overall amount of cadmium in the sensitized film of <0.5 atomic %. The extremely low content of Cd in these devices significantly reduces concerns of potential toxicity relative to the already widely used CdTe thin-film solar cells. After Cd-treated QDs are recapped with short ligands (chosen from those in Fig. 3a ), they are incorporated into a mp-TiO 2 photoanode via soaking in dilute QD–octane or methanol solutions. We found that the identity of the ligand had a major impact on device performance. We observe that tert -butylamine (tBA), n -butylamine (nBA) and sec -butylamine (sBA) are equally effective at achieving high QD-loading according to optical absorption measurements ( Fig. 3b ). Unlike most QDSSC reports, we achieve this high degree of loading (using butylamine) by direct attachment without the assistance of a high electric field (electrophoretic deposition) [27] or bifunctional linkers (for example, MPA) [25] . On the other hand, the use of the native ligands (oleylamine and DDT), mercaptoproprionic acid (MPA) or pyridine resulted in much poorer loading. Accordingly, we found that the choice of the ligand did not affect V oc , but did have a significant effect on J sc ( Fig. 3d and Supplementary Table S4 ). Typically, improvement in only J sc would indicate that enhanced light-harvesting is the primary reason for the benefit of using the butylamines, rather than a reduction in recombination losses, which would be expected to impact V oc as well. However, in liquid-junction cells the absorber band-gap (that is, QD band-gap) can be well in excess of the maximum attainable V oc , which is determined by the energy difference between the TiO 2 Fermi level and the redox potential of the electrolyte. In this case, the relationship between recombination, open-circuit voltage and short-circuit current is not as trivial as with solid-state solar cells, and so we can’t fully rule out differences in recombination using these ligands. In fact, we do observe differences in the absorption-normalized PL intensity ( Fig. 3c ) from QDs recapped with these ligands in solution (prior to sensitization), which indicates differences in non-radiative recombination related to surface traps. Therefore, in addition to differences in loading, J sc may also be impacted by non-radiative recombination within the QD absorbers. At this time we do not have a complete understanding of why sBA and nBA show poorer performance than tBA, but we note that the lower PL intensity ( Fig. 3c ) from QDs recapped with these isomers may implicate recombination as a factor. Furthermore, we find that devices made using QDs recapped with nBA show a surprisingly poor stability (blue curves on Fig. 3e ) compared with sBA and tBA, which could also be related to the particular ineffectiveness of nBA at surface-trap passivation. 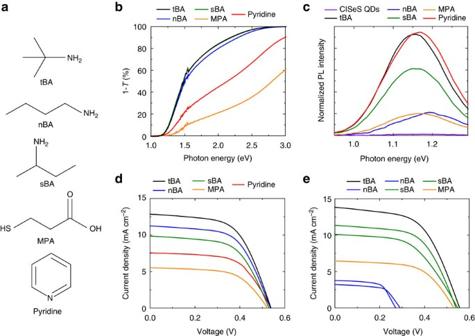Figure 3: Organic passivation of QDs. (a) Molecular structures of ligands investigated in this work. (b) The absorbed fraction of incident radiation (as 1−T, whereTis film transmittance in %) of sensitized films using identical QDs recapped with various ligands. Contributions from absorption/scattering by the glass/FTO/mp-TiO2substrate have been subtracted in each case; a scattering layer was not used for these measurements. (c) Absorption-normalized PL in solution of as-synthesized CISeS QDs (purple) and cation exchanged (Cd-OA 50 °C treatment) after recapping with each ligand. (d) Current density versus voltage characteristics for each ligand 5 days after fabrication. (e) Performance of the QDSSCs after 60 days. Two devices are shown for the nBA (blue) and sBA (green) cases to demonstrate the reproducibility of the result. tBA is shown to have the highestJscinitially and after a period of months. These devices did not have the mp-TiO2scattering layer nor a ZnS SILAR coating. The devices fabricated with pyridine-capped QDs failed after roughly 2 weeks. The photovoltaic performance properties related todandecan be found inSupplementary Tables S4 and S5. Figure 3: Organic passivation of QDs. ( a ) Molecular structures of ligands investigated in this work. ( b ) The absorbed fraction of incident radiation (as 1− T , where T is film transmittance in %) of sensitized films using identical QDs recapped with various ligands. Contributions from absorption/scattering by the glass/FTO/mp-TiO 2 substrate have been subtracted in each case; a scattering layer was not used for these measurements. ( c ) Absorption-normalized PL in solution of as-synthesized CISeS QDs (purple) and cation exchanged (Cd-OA 50 °C treatment) after recapping with each ligand. ( d ) Current density versus voltage characteristics for each ligand 5 days after fabrication. ( e ) Performance of the QDSSCs after 60 days. Two devices are shown for the nBA (blue) and sBA (green) cases to demonstrate the reproducibility of the result. tBA is shown to have the highest J sc initially and after a period of months. These devices did not have the mp-TiO 2 scattering layer nor a ZnS SILAR coating. The devices fabricated with pyridine-capped QDs failed after roughly 2 weeks. The photovoltaic performance properties related to d and e can be found in Supplementary Tables S4 and S5 . Full size image The overall device performance ( Fig. 3d ) and longevity ( Fig. 3e ) were optimal with tBA. Relatively high band-edge PL quantum yield (QY) from tBA-capped QDs in solution (~20%, Supplementary Table S1 ) suggests that recapping with tBA is also effective at passivating surface traps, in addition to improving QD-loading and stability. Indeed, our observations confirm what others have reported: that effective organic passivation in combination with robust inorganic passivation is critical for high-performance QD PVs [3] , [34] . At the same time, the small length of the tBA ligand enables efficient electron extraction into TiO 2 by allowing relatively intimate contact between QDs and the TiO 2 surface ( Fig. 4a ). Full understanding of the mechanism of initial attachment requires further study, but may be related to QD charging (electrostatic attraction to induced charges); however, once contact is made, Van-der-Waals forces and insolubility of the QDs in the electrolyte are likely to be the primary reasons for their robust and prolonged attachment to the mp-TiO 2 . 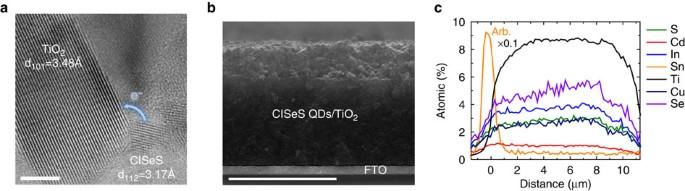Figure 4: QD loading. (a) TEM image of a QD/TiO2heterojunction showing the intimate contact between them when tBA is used as a ligand. Scale bar, 5 nm. (b) SEM cross-sectional image of our champion device. The substrate used was fluorinated tin oxide (FTO)-coated glass. Scale bar, 10 μm. (c) EDX spectroscopy line scan of the cross-section showing the elemental composition of the sensitized film. Atomic percentages are of the total composition excluding oxygen (not shown) and tin (shown in orange, but arbitrarily scaled), and the titanium atomic percent is scaled down by a factor of 10 for ease of comparison. Figure 4: QD loading. ( a ) TEM image of a QD/TiO 2 heterojunction showing the intimate contact between them when tBA is used as a ligand. Scale bar, 5 nm. ( b ) SEM cross-sectional image of our champion device. The substrate used was fluorinated tin oxide (FTO)-coated glass. Scale bar, 10 μm. ( c ) EDX spectroscopy line scan of the cross-section showing the elemental composition of the sensitized film. Atomic percentages are of the total composition excluding oxygen (not shown) and tin (shown in orange, but arbitrarily scaled), and the titanium atomic percent is scaled down by a factor of 10 for ease of comparison. Full size image As inferred from energy-dispersive X-ray (EDX) spectroscopy measurements of photoanode cross-sections ( Fig. 4b ), the use of this ligand results in QD/TiO 2 films with highly uniform loading throughout the mp-TiO 2 ( Fig. 4c ). By comparing QD constituents (for example, Cu, In, Se, S) to measured meso-porous support content (Ti), we estimate that ~3% of the solid material (by atomic %) in the film is QD material. The fraction of QDs is reduced near the top of the film where a scattering layer of 400 nm TiO 2 particles (presenting a lower surface area for attachment [28] ) is added prior to sensitization to improve light harvesting, which is consistent with SEM cross-section images showing the larger pores in the scattering layer are not filled with aggregated QDs. Investigation of the methanol-based polysulfide electrolyte Following electron transfer from a QD to the TiO 2 ( Figs 1c and 4a ), the photogenerated hole is reduced by the electrolyte, which also serves as a hole transporting medium. In order to elucidate the importance of electrolyte parameters, we explored dilution of the electrolyte with methanol [26] , [35] . Zewdu et al. [35] reported a synergistic effect of methanol in combination with a ZnS SILAR treatment of CdSe/CdS-sensitized TiO 2 , which was preliminarily attributed to improved wetting of the photoanode by the electrolyte. In our experiments, we observe a significantly greater improvement in the PV performance upon addition of methanol than previously seen. Specifically, as the aqueous polysulfide electrolyte (2 M Na 2 S and 2 M S) is diluted with methanol ( Fig. 5a ), the measurements of current–voltage ( J–V ) characteristics indicate a greatly increased photocurrent and a reduced series resistance ( R series , determined as the inverse of the slope of the J–V curve at the V oc ), which leads to a higher FF. Reduced R series is likely due to the lower viscosity of methanol (0.54 mPa s) relative to water (0.89 mPa s), enabling faster ionic transport (ionic mobility increases with decreasing solvent viscosity). The enhancement in the photocurrent however can be caused by several effects. In our studies, we have considered three possibilities: (1) methanol can potentially act as a sacrificial electron donor aiding in the reduction of photogenerated holes [26] , [27] ; (2) it could improve electron injection efficiency by lowering the Fermi level of the TiO 2 film [36] and (3) it can lead to better contact between the QDs and the electrolyte due to improved wetting [35] . 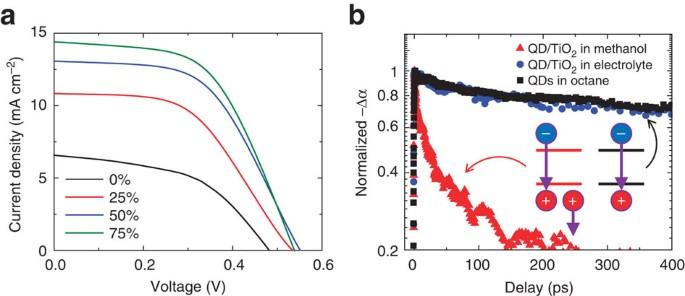Figure 5: Dependence of device performance on the electrolyte composition. (a) Current density versus voltage characteristics under simulated sunlight for QDSSCs with varying amounts of methanol in the electrolyte (reducing the polysulfide concentration by dilution). A ZnS SILAR coating was not used. A table of the photovoltaic performance properties can be found inSupplementary Table S6. (b) QD population decay monitored by probing the temporal evolution of the band-edge bleach with transient absorption. The traces in the figure correspond to isolated QDs dispersed in octane (black square), and QDs attached to the TiO2matrix exposed to either methanol (red triangle) or electrolyte (blue circle). Figure 5: Dependence of device performance on the electrolyte composition. ( a ) Current density versus voltage characteristics under simulated sunlight for QDSSCs with varying amounts of methanol in the electrolyte (reducing the polysulfide concentration by dilution). A ZnS SILAR coating was not used. A table of the photovoltaic performance properties can be found in Supplementary Table S6 . ( b ) QD population decay monitored by probing the temporal evolution of the band-edge bleach with transient absorption. The traces in the figure correspond to isolated QDs dispersed in octane (black square), and QDs attached to the TiO 2 matrix exposed to either methanol (red triangle) or electrolyte (blue circle). Full size image The first possibility can be excluded based on the prolonged stability of our device performance achieved without replenishing methanol in the electrolyte, which would be impossible if methanol served as a sacrificial donor. Furthermore, we observe in a control study that the PL QY from QD-sensitized films immersed in water or methanol without electrolyte is more than two orders of magnitude lower than that of the same films with electrolyte ( Supplementary Table S1 ). Similar observations have been made in DSSCs where dye molecules remain oxidized for orders of magnitude longer timescales in the absence of a redox electrolyte [37] , [38] . This result suggests that in pure methanol, holes are not removed from the QDs, which leads to a build-up of a net positive charge in photo-excited QDs and associated activation of a fast non-radiative decay channel via Auger recombination of charged excitons [39] , [40] . This assessment is confirmed by transient absorption (TA) studies of carrier dynamics in QD-sensitized films upon their exposure to various solvents ( Fig. 5 b). In the case of dry methanol, the decay is dominated by a fast 20–50 ps component, which is consistent with Auger recombination of a positively charged exciton (positive trion), a process in which the electron-hole recombination energy is transferred to a pre-existing hole [39] , [41] (left inset in Fig. 5b ). This suggests that the hole remaining in the QD following electron transfer to TiO 2 is not reduced by methanol in the absence of electrolyte and still remains in the QD when it absorbs the next photon. On the other hand, the QD hole is efficiently regenerated in the presence of electrolyte: the measured dynamics are nearly identical to those of isolated QDs dispersed in solution, which is dominated by recombination of neutral excitons (right inset in Fig. 5b ). We also observe a less pronounced ~400 ps decay component in methanol that we attribute to surface traps that are effectively passivated by the electrolyte. Further, these TA measurements conducted on samples exposed to electrolyte also provide a lower limit for the characteristic time of electron transfer of >5 ns, which is surprisingly long compared with some previous reports on photo-excited dynamics at QD-metal oxide interfaces [27] , [42] . However, this long time scale is consistent with our observation that various types of QD surface modification lead to correlated changes in QD PL emission efficiency and their performance in PV devices. These correlations would not have been observed if electron transfer was significantly faster than competing recombination mechanisms in isolated QDs. Next, we analyse the potential effect of methanol on the Fermi level of TiO 2 . It is known that methanol can modify TiO 2 surface structure [43] or undergo photochemical reactions in the presence of a catalyst [44] . Reactions between TiO 2 and methanol could increase photocurrent yield if they lead to a lowering of the TiO 2 Fermi level (that is, if TiO 2 is oxidized as a result of the reaction), as this would make electron injection from QDs even more favourable. In order to see the effects of intentional oxidation of a TiO 2 anode, we use Li + ions that are known to effectively remove electrons from the surface of TiO 2 (ref. 37 ). This approach has been utilized to realize ~100% electron injection efficiency in CdSe-QDSSCs [36] . When we add Li 2 S to the electrolyte at 50% methanol concentration, we do indeed observe an increase in J sc ; however, it is accompanied by a reduction in the V oc ( Supplementary Fig. S6 and Supplementary Table S7 ). Both of these are anticipated results of a lower TiO 2 Fermi level, which in addition to increasing J sc should also reduce the energy offset between the anode Fermi level and the electrolyte redox potential, decreasing V oc . If methanol were also oxidizing TiO 2 , then we would expect V oc to be reduced with increasing methanol content, which is not observed; in fact, increasing amounts of methanol, if anything, lead to higher V oc ( Fig. 5a ). Finally, we analyse the third possibility, namely that improved wetting of the QD/TiO 2 surface by the methanolic electrolyte solution can facilitate hole extraction from the QDs and thus improve J sc . The degree of wetting of a solid material by a liquid depends on the relative surface tensions of the three joining interfaces (that is, γ gas–liquid , γ gas–solid , γ liquid–solid ). As the electrolyte solvent changes from water to methanol, only the two tensions involving the liquid will be modified. Estimating the surface tension of mp-TiO 2 /QDs with various solvents (that is, γ liquid–solid ) in an actual device is complicated by the high surface/volume ratio [45] , the hydrophobicity of the ligand-passivated QD surfaces within the sensitized film, and by dramatic changes in wetting behaviour (TiO 2 becomes amphiphilic) under ultra-violet irradiation [46] . However, a comparison of the well-established surface tensions between air and most solvents (that is, γ gas–liquid ), can be instructional in this case. The three-fold greater surface tension at a water–gas interface ( γ air–water =72 mN m −1 ) than at a methanol–gas interface ( γ air–methanol =23 mN m −1 ) means that methanol wets most surfaces better than water. In a simple test of placing a droplet of both solvents on a mp-TiO 2 film, methanol clearly demonstrated a greater tendency to wet the surface ( Supplementary Fig. S5 ). As photocurrent relies directly on contact between the electrolyte and the QD surface (for hole extraction), our observations of increased J sc are consistent with improved wetting by the electrolyte. Meso-textured Cu x S cathode Another critical element of a sensitized solar cell is the cathode, which has a significant effect on the overall device performance through its influence on R series and thus FF. In our solar cells we employ a Cu x S cathode ( Fig. 6 ), which allows us to obtain R series of 10 Ω·cm 2 and FF of ~0.60 in the best devices, among the highest for QDPVs. Our simple method for making the cathode is by chemical transformation of 100-nm thick thermally evaporated Cu (on FTO) by exposure to the polysulfide electrolyte. Based on EDX measurements, the Cu x S has an x =1.0 stoichiometry upon fabrication (that is, covellite, a p- type metal), but it becomes sulphur enriched ( x of ca . 0.8) after being used in a device. The observed level of relative copper deficiency corresponds to an even higher degree of p -type doping, which should greatly improve cathode conductivity. Further, after sulphurisation our cathodes develop a meso-textured structure, characterized by a large surface area ( Fig. 6b inset), which persists after many months of testing ( Supplementary Fig. S4 ) and facilitates charge collection from the electrolyte. Together with improved conductivity, this is likely a second major factor in reduced R series and improved performance in our devices compared with previously published studies typically with Cu 2 S, which is a semiconductor. To better understand the contribution of the cathode and other factors (for example, charge-transfer resistance, electrolyte, mp-TiO 2 ) to the aggregate series resistance of the device (measured by the inverse slope of the J–V curve), impendence spectroscopy may be insightful. 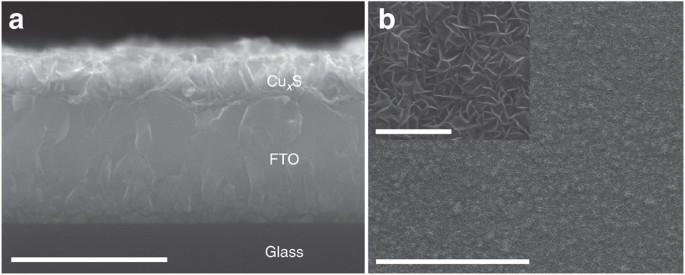Figure 6: CuxS cathode. (a) SEM image of a cross-section of a fresh glass/FTO/CuxS cathode wherex=1.0 according to EDX analysis. Scale bar, 1 μm. (b) SEM image from the top-down perspective of the cathode. Scale bar, 10 μm. Higher magnification inset shows the flower-like structures with high surface area. Scale bar, 1 μm. Figure 6: Cu x S cathode. ( a ) SEM image of a cross-section of a fresh glass/FTO/Cu x S cathode where x =1.0 according to EDX analysis. Scale bar, 1 μm. ( b ) SEM image from the top-down perspective of the cathode. Scale bar, 10 μm. Higher magnification inset shows the flower-like structures with high surface area. Scale bar, 1 μm. Full size image QDSSC stability and certification A common and critical issue with QDSSCs is their poor stability resulting from electrochemical corrosion of many candidate sensitizers [23] , [47] . As our QDs are synthesized under excess sulphur conditions, we expected that our CISeS QDs would be chemically stable in the presence of the sulphur-based electrolyte. However, as we added more Se to reduce the band-gap of the QDs, they became less stable in the electrolyte, probably due to the replacement of Se by S anions at the surface over time [24] . The chemical incompatibility problem is typically addressed in the QDSSCs by the application of a thin insulating ZnS layer deposited by SILAR. The partial cation exchange (with Cd 2+ or Zn 2+ ) of QDs in our devices prior to sensitization (discussed earlier) helps solve the stability issue, and allows for stable operation of the devices for 1–2 months instead of 1–2 days [24] . To further improve the stability, we deposit two monolayers of ZnS using SILAR on photoanodes after they are sensitized with Cd-treated and tBA-recapped CISeS QDs. Following this procedure, the initial performance of a device is unchanged. However, the thin layer of ZnS seems to act as a good chemical barrier, which complements the existing barrier due to cation exchange without appreciably suppressing hole extraction into the electrolyte (ZnS deposited by SILAR is not expected to influence electron extraction, as the QD-TiO 2 close contacts are established prior to ZnS application). Devices with the ZnS SILAR consistently showed prolonged stability under air exposure ( Fig. 7a ), although it is worth noting that even without the ZnS layer, some devices survived for up to 2 months ( Fig. 3e ). This is in drastic contrast to previously reported high-performance QDSSCs that were stable for just a few minutes [23] . The eventual catastrophic failure of the devices with a ZnS SILAR coating was associated with electrode delamination (for example, Cu x S would peel off the substrate), which can be addressed by establishing better adhesion between layers during electrode fabrication. In order to better elucidate the true long-term stability of these devices, extended light-soaking tests should be conducted. Studies of the effect of light-soaking for 30 h indicate that the performance of our devices improves over the first ~15 min, which we attribute to improved ionic transport due to heating of the electrolyte, and then stays unchanged once the device temperature stabilizes under the light source ( Supplementary Fig. S8 ). 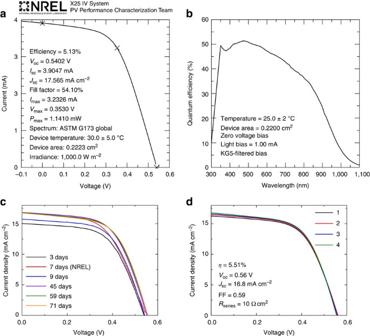Figure 7: Certified PV performance and stability. (a) Current density versus voltage characteristics of a QDSSC certified by NREL. (b) EQE spectra for the device measured at NREL. (c) Performance of our champion device (different from the one inaandb) over time, including the certification data from NREL. The device was tested further (for example, day 1, day 4, day 6, and so on), but these measurements are not included in for plot clarity. (d) Sequential measurements of our champion device at 71 days under constant illumination for ~15 min. Each measurement takes 90 s, there was a 1 min delay betweenJ–Vmeasurements. The photovoltaic performance properties related tocanddcan be found inSupplementary Tables S8 and S9. Figure 7: Certified PV performance and stability. ( a ) Current density versus voltage characteristics of a QDSSC certified by NREL. ( b ) EQE spectra for the device measured at NREL. ( c ) Performance of our champion device (different from the one in a and b ) over time, including the certification data from NREL. The device was tested further (for example, day 1, day 4, day 6, and so on), but these measurements are not included in for plot clarity. ( d ) Sequential measurements of our champion device at 71 days under constant illumination for ~15 min. Each measurement takes 90 s, there was a 1 min delay between J–V measurements. The photovoltaic performance properties related to c and d can be found in Supplementary Tables S8 and S9 . Full size image The stability of our devices enabled us to have two of them (one with and one without a ZnS SILAR coating) certified by the PV Characterization Team at the National Renewable Energy Laboratory (NREL) 1 week after fabrication. Both devices were certified at 5.1% and the details of the certified performance can be found in Fig. 7a (device without ZnS) and in the Supplementary Fig. S2 (device with ZnS). As far as we know, these are the only certified performances reported for any QDSSC, which is important for a variety of reasons (see Supplementary Discussion ). We continued testing the certified device, which had a ZnS SILAR coating periodically, with storage under ambient but dark conditions ( Fig. 7c ). This device survived 71 days, and maintained an efficiency of 5.5% through the final measurement using our in-house solar simulator under continuous illumination ( Fig. 7d and Supplementary Table S9 ), which is the highest reported for any colloidal (that is, non-SILAR) QDSSC. Interestingly, the NREL-certified photocurrent was ~10% (relative) higher in this device than what we measured with our solar simulator, indicating that our 5.5% record measurement may be slightly underestimating the performance. Compared with a maximum possible EQE of ~80% (considering absorption and reflection losses due to the fluorinated tin oxide on glass electrode), our best devices achieve a peak EQE of ~60% at ~3.0 eV, although it is considerably lower for lower-energy photons ( Fig. 7b ). The relatively low and non-flat EQE of our devices suggests that there is significant room for improvement of J sc by enhancing absorption (for example, via improved QD-loading) and/or by optimizing internal charge collection efficiencies (for example, via faster charge extraction). Although we observe relatively high QD-loading by simply soaking the electrode in a dilute solution of (recapped) QDs, loading might be further improved by the use of electrophoretic deposition [27] , [48] or by attachment using alternative bifunctional linkers [25] , [49] . In summary, we have shown that QDSSCs can exhibit both high performance and high stability using low-toxicity materials and low-cost fabrication methods. We have identified optimal conditions for the sensitization of mp-TiO 2 with CISeS QDs using a very mild cation exchange with Zn 2+ or Cd 2+ followed by washing/recapping with tBA. Addition of a ZnS layer by SILAR does not lead to enhanced efficiency but further improves device stability. Adding methanol to the electrolyte significantly enhances the device performance by increasing photocurrent and lowering series resistance. We demonstrated a nanostructured Cu x S (where x <1.0) cathode can be made by a simple low-cost method, and acts as an extremely effective reducing catalyst for the polysulfide electrolyte and enabled us to achieve series resistances on par with the best DSSCs that use platinum. Recognizing the challenges in accurately characterizing PVs, and thus the difficulties in comparing between various published results, we report the first certified performance of a QDSSC at 5.1% efficiency. Our champion efficiency approaches the highest reported values for any type of QD solar cells, yet our devices do not degrade for months even if stored in air: this is orders of magnitude longer than in any previous report on QD PVs. Given the fairly low EQEs even in our record devices, we expect that with further optimization, the performance of these novel PV devices can be enhanced considerably, making them competitive with well-established dye-sensitized solar cells. Synthesis of CISeS QDs CISeS QDs were synthesized via a modification of the Li et al. [30] method [24] . Typically, 1 mmol of copper iodide and 1 mmol of indium acetate are dissolved in 5 ml of 1-dodecanethiol and 1 ml of oleylamine, and the mixture is degassed under vacuum in a 50 ml flask at 100 °C for 30 min. The solution was heated to 130 °C until it became yellow and transparent, and then degassed again for 30 min at 100 °C. The flask is then slowly heated to a growth temperature of 230 °C, but at a temperature of 220 °C, slow injection of 6 mmol of 2 M TOP-Se (~12 ml h −1 ) begins. After 30 min the reaction was cooled and the QDs were cleaned by dissolving in chloroform and precipitation with methanol. The precipitated QDs were collected by centrifugation and the supernatant was discarded. The QDs were stored in 5 ml of octane or ODE following cleaning. The synthesis typically results >90% chemical yield of QDs (relative to the copper and indium precursors). Cation exchange and recapping of QDs For cation exchange with Cd 2+ or Zn 2+ , a stock solution of 0.5 M cadmium or zinc oleate was prepared with 3:1 oleic acid:Cd/Zn dissolved in ODE. 4 ml of the cleaned QDs in ODE solution (~50 mg ml −1 ) were added to 4 ml of 0.5 M Cd or Zn-oleate solution and the temperature was set to 50–150 °C for 10 min depending on the desired degree of cation exchange. Following cation exchange, the reaction solution was dissolved in chloroform, and then acetone was added to precipitate the QDs. The precipitated QDs were collected by centrifugation, and then dissolved in chloroform. Ligand exchange of QDs Following cation exchange and purification of QDs, methanol was added to precipitate the QDs from chloroform. Precipitated QDs were collected by centrifugation and the supernatant was discarded. For tBA, nBA, sBA and pyridine recapping, the ligand was used as a solvent to dissolve the precipitated QDs with sonication used to speed up dissolution and recapping. Then, methanol was added to precipitate the QDs, which were collected by centrifugation and the supernatant was discarded. The ligand was again used as a solvent to dissolve the precipitated QDs and these solutions were sonicated for a few minutes at room temperature. Methanol was added to precipitate the QDs, which were collected by centrifugation. The above process was optimized to give the highest QD-loading in the mp-TiO 2 film for tBA-capped QDs. The optimal conditions may be different for the other ligands. Longer exposure of the QDs to the new ligands or heating during exposure might give more complete recapping, but resulted in poorer loading, probably due to partial aggregation of QDs during recapping. The recapped QDs were dissolved in octane (~0.05 g ml −1 ), and the solution was centrifuged to remove large aggregates that occasionally formed during recapping. Any precipitate was discarded. The QD–octane supernatant was diluted with octane to an optical density of ~0.2 (~0.01 g ml −1 ) at the 1S absorption peak (typically 850 nm), and used to prepare QD-sensitized mp-TiO 2 films. For MPA recapping, the QDs were recapped by dissolving precipitated QDs in a mixture of 1:1 chloroform and MPA, then precipitating by adding methanol, and centrifuged. The supernatant was discarded, and the QDs were dissolved in the same total volume of MPA and methanol (1:1). The solution was sonicated for a few minutes. Chloroform was added to precipitate the MPA-capped QDs, and the QDs were collected by centrifugation. The MPA-capped QDs were dissolved in methanol (~0.05–0.1 g ml −1 ), and the solution was centrifuged to remove aggregates that formed during recapping and to remove partially recapped QDs. The QD–methanol supernatant was diluted with methanol to an absorbance of about 0.2 (~0.01 g ml −1 ) at the 1S absorption peak (typically 850 nm), and used to prepare QD-sensitized mp-TiO 2 films. Fabrication of QDSSCs Scattering and non-scattering mp-TiO 2 films are prepared by automated, iterative screen-printing (LS-150, New Long Seimitu Kogyo Co.) of TiO 2 pastes containing ~20 nm and ~400 nm TiO 2 particles, respectively, on fluorinated tin oxide (FTO)-coated glass. A dense blocking layer of TiO 2 is not used. The α-terpineol based pastes are fired at 500 °C for 1 h under air. The 8 μm (or 13 μm with the scattering layer) thick mp-TiO 2 films are sensitized by soaking in dilute QD–octane solutions for 36 h. The films were then rinsed with octane (or methanol for MPA-capped QDs) to remove unattached QDs. The cathode is fabricated by thermally evaporating 100 nm of Cu onto a FTO-coated glass substrate, and subsequent immersion in an aqueous polysulfide electrolyte (aqueous 1 M Na 2 S plus 1 M S) for 15 min to form Cu x S/FTO. The device is completed by sandwiching the electrodes around a 40–50 μm Surlyn spacer (DuPont) and sealing by heating the polymer frame. Unless otherwise noted, the devices are filled with the polysulfide electrolyte composed of 1 M Na 2 S and 1 M S in methanol and water (1:1). For champion devices, silver paint and Cu wires was added to the contacts. The device active area is defined by a 0.47 cm by 0.47 cm (that is, 0.2209, cm 2 ) black metal aperture, which is slightly smaller than the mp-TiO 2 area. The mp-TiO 2 scattering layer was only used for champion devices that were certified. As our device active area is relatively large we do not see significant device to device variations. However, we fabricated two devices for each case to confirm that any trends we observe are real. Duplicates of all devices were fabricated and tested for consistency and if the performance varied by >5% we repeated the study. Transmission electron microscopy TEM samples were prepared from a dilute solution of NCs in chloroform drop-cast onto Cu grids (obtained from Ted Pella) with a thin carbon film on a holey carbon support. TEM analysis was carried out with a JEOL 2010 TEM operating at 200 kV. Scanning electron microscopy and X-ray dispersive spectroscopy SEM samples were prepared by breaking a QDSSC anode or cathode in half. The SEM used a Quanta 400 field emission gun made by FEI Company. The 20 kV electron beam was scanned across the cross-section, and then the energy and the count of X-rays were measured. Elemental analysis was conducted using Genesis EDX software. Optical absorption and photoluminescence spectroscopy All optical measurements of QDs in solution were performed in either chloroform or octane using a quartz cuvette. UV–vis absorption spectra were obtained with Agilent 8453 photodiode array spectrometer. PL measurements were performed using home-build spectrofluorimeter consisting or 808 nm excitation diode laser, a liquid nitrogen-cooled InSb detector and a grating monochromator. The excitation beam was mechanically chopped at 3 kHz and the signal was measured using a lock-in amplifier. For PL quantum yield (QY) measurements, optically dilute samples were magnetically stirred and the QY values were measured using relative technique by comparing integrated PL intensities to an IR-26 dye standard. The spectra were corrected for the wavelength-dependence sensitivity of the system. Solar cell characterization A class ABA solar simulator (AM 1.5 G), built by PV Measurements, calibrated using a Newport-certified single crystal Si solar cell, was used to irradiate the QDSSCs during I – V measurement (in-house). The voltage was swept from −0.1 to 0.6 V at 0.01 V per step with a 1 s delay-time prior to measurement and 200 ms collection time at each point. A square black mask (0.2209, cm 2 ) was attached to the solar cells to precisely define the active area of the device. An additional black cardboard mask (~5 cm by 5 cm outer edges) was placed on top of the contacted device (masking area outside the 0.2209, cm 2 mask) immediately prior to current–voltage measurement to prevent scattering of light into the device by the contacting alligator clips. For continuous illumination testing, devices were shorted in between measurements. How to cite this article: McDaniel, H. et al. An integrated approach to realizing high-performance liquid-junction quantum dot sensitized solar cells. Nat. Commun. 4:2887 doi: 10.1038/ncomms3887 (2013).